β-lactam antibiotics promote bacterial mutagenesis via an RpoS-mediated reduction in replication fidelity Regardless of their targets and modes of action, subinhibitory concentrations of antibiotics can have an impact on cell physiology and trigger a large variety of cellular responses in different bacterial species. Subinhibitory concentrations of β-lactam antibiotics cause reactive oxygen species production and induce PolIV-dependent mutagenesis in Escherichia coli . Here we show that subinhibitory concentrations of β-lactam antibiotics induce the RpoS regulon. RpoS-regulon induction is required for PolIV-dependent mutagenesis because it diminishes the control of DNA-replication fidelity by depleting MutS in E. coli, Vibrio cholerae and Pseudomonas aeruginosa. We also show that in E. coli , the reduction in mismatch-repair activity is mediated by SdsR, the RpoS-controlled small RNA. In summary, we show that mutagenesis induced by subinhibitory concentrations of antibiotics is a genetically controlled process. Because this mutagenesis can generate mutations conferring antibiotic resistance, it should be taken into consideration for the development of more efficient antimicrobial therapeutic strategies. For each new antibiotic, a countdown begins until the inevitable clinically significant resistance arises. There is growing evidence that de novo antibiotic resistance can emerge at low antibiotic concentrations [1] , [2] , [3] . Understanding the molecular mechanisms that are involved in the emergence of resistance in a bacterial population at low antibiotic concentrations is therefore of major importance. Low concentrations of different classes of antibiotics are frequently encountered environmental cues to which bacteria must respond appropriately to maintain fitness [4] , [5] . During therapeutic use in humans and animals, as well as during growth promotion use in animals, bacteria face wide gradients of antibiotic concentrations in highly compartmentalized host bodies [7] . In addition, 30–90% of ingested antibiotics are excreted unchanged from human and animal bodies via urine and faeces and, as a result, contaminate water and soil [8] , [9] , [10] . Subinhibitory concentrations of antibiotics, regardless of their targets and modes of action, provoke considerable changes in transcription and trigger a wide variety of cellular responses in different bacterial species [6] , [11] . For example, subinhibitory concentrations of antibiotics induce the expression of virulence genes, such as toxins and adhesins in Escherichia coli and Staphylococcus aureus [12] , [13] . Low concentrations of streptomycin and norfloxacin induce genetic transformability in Streptococcus pneumonia , and thus facilitate the acquisition of antibiotic resistance through horizontal gene transfer [14] . Similarly, low concentrations of antibiotics induce mutagenesis in Pseudomonas aeruginosa [15] , S. pneumoniae [16] , E. coli [2] , Vibrio cholerae [17] and S. aureus [2] . For E. coli and S. aureus , the increased formation of reactive oxygen species (ROS) induced by antibiotics is proposed to be the critical step in antibiotic-induced mutagenesis [2] . The aim of the present study is to understand whether subinhibitory concentrations of antibiotics also induce the general stress response that is mediated by the alternative sigma factor RpoS (σ S ) [18] . This stress response is induced by a wide variety of stresses [18] . The induction of the RpoS regulon is subjected to complex regulation at all levels of gene expression, that is, transcription, translation and protein stability [18] . The induction of this regulon results in changes in the expression of hundreds of genes involved in the modulation of membrane permeability, cell shape, cellular metabolism and the capacity to protect and repair cellular macromolecules, as well as the expression of virulence genes. The induction of this regulon allows bacterial cells to enter into a multiresistant state. The induction of the RpoS regulon was reported to be required for carbon source starvation-induced mutagenesis in E. coli , largely due to the induction of the dinB gene [19] , [20] , [21] . This gene, which is also regulated by the LexA SOS repressor, codes for the error-prone DNA polymerase IV (PolIV). This specialized DNA polymerase was previously described as an essential factor in the cytotoxic and mutagenic property of bactericidal antibiotics [22] . PolIV was shown to incorporate mutagenic oxidized nucleotides that are generated during antibiotic treatment [22] , [23] , which could explain why this polymerase promotes mutations in ceftazidime-treated E. coli cells [24] . For this reason, we also investigated whether the mutagenesis induced by subinhibitory concentrations of antibiotics could be regulated by RpoS via induction of the dinB gene or/and modulating the expression of other genes. We found that the RpoS regulon is induced by subinhibitory concentrations of bactericidal antibiotics belonging to different families, such as quinolones, aminoglycosides and β-lactams. Furthermore, we showed that the induction of this regulon is required for PolIV-dependent mutagenesis because it diminishes control of the DNA-replication fidelity by downregulating mismatch repair in E. coli, V. cholerae and P. aeruginosa. In E. coli , we discovered that the decrease in mismatch-repair activity depends on the RpoS-controlled small RNA, SdsR, which seems to directly repress the mutS mRNA. SdsR is the first small RNA to be involved in the response to antibiotics. Induction of the general stress response by antibiotics To monitor the induction of the general stress response, we constructed a p ada :: lac reporter fusion ( Supplementary Methods ). The Ada protein regulates the adaptive response to alkylating agents [25] . In the absence of alkylation DNA damage in growing cells, Ada negatively regulates its own transcription [26] . Upon DNA alkylation, the Ada protein is converted into a transcriptional activator that promotes its own transcription, as well as that of several others genes involved in the repair of mutagenic and cytotoxic alkylation DNA damages [27] . In stationary-phase cells, RpoS upregulates the ada gene expression independent of the presence of the Ada protein in the absence of alkylation DNA damage [28] . The advantage of using the p ada :: lac fusion as a reporter for the RpoS-regulon induction is that ada gene expression is known to be dependant only on Ada and RpoS, which is not the case for many of the RpoS-regulated genes that are frequently regulated by several independent regulators [29] , [30] . As expected, the induction of the p ada :: lac reporter by alkylating agents was Ada-dependent and RpoS-independent, and its induction in stationary-phase cells depended exclusively on RpoS ( Fig. 1 and Supplementary Fig. S1 ). We used this reporter fusion to investigate the induction of the RpoS regulon by different antibiotics using disk diffusion assays on LB plates supplemented with X-gal. Induction was visualized as a blue ring close to the growth-inhibition zone. Bactericidal antibiotics, such as quinolones, aminoglycosides and β-lactams, induced the RpoS regulon ( Fig. 1 , Supplementary Fig. S1 and Supplementary Table S1 ). 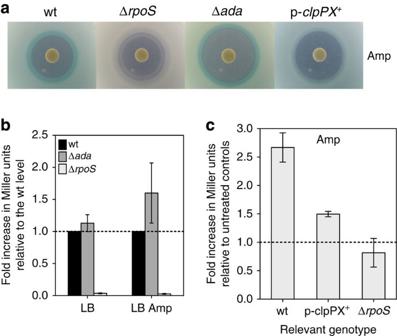Figure 1: Monitoring induction of the RpoS regulon using the pada::lacZreporter fusion. Induction was visualized as blue rings using a disk diffusion assay on LB plates supplemented with X-gal (a) and by quantifying β-galactosidase activity in liquid LB medium (b,c). (b) Wild-type (wt), Δadaand ΔrpoSstrains grown in LB and LB supplemented with 1 μg ml−1of ampicillin (Amp) (LB Amp). For each genotype, the fold increase relative to the wt level for each experimental condition is presented. (c) wt, wt strain overexpressing the ClpP–ClpX complex and the ΔrpoSstrain grown in LB supplemented with 1 μg ml−1of ampicillin. For each genotype, the fold increase relative to the untreated control is presented. For all measures, each point represents the mean±s.e.m. of three independent experiments. Figure 1: Monitoring induction of the RpoS regulon using the p ada :: lacZ reporter fusion. Induction was visualized as blue rings using a disk diffusion assay on LB plates supplemented with X-gal ( a ) and by quantifying β-galactosidase activity in liquid LB medium ( b , c ). ( b ) Wild-type (wt), Δ ada and Δ rpoS strains grown in LB and LB supplemented with 1 μg ml −1 of ampicillin (Amp) (LB Amp). For each genotype, the fold increase relative to the wt level for each experimental condition is presented. ( c ) wt, wt strain overexpressing the ClpP–ClpX complex and the Δ rpoS strain grown in LB supplemented with 1 μg ml −1 of ampicillin. For each genotype, the fold increase relative to the untreated control is presented. For all measures, each point represents the mean±s.e.m. of three independent experiments. Full size image For a more detailed study of the impact of the RpoS-regulon induction on cell physiology, we chose the β-lactam antibiotic ampicillin as a model drug. The reporter induction by ampicillin was Ada-independent and RpoS-dependent in the disk diffusion assay, as well as in liquid medium supplemented with 1 μg ml −1 of ampicillin. This concentration of ampicillin, which is 50% of the minimum inhibitory concentration (MIC) as defined for all the E. coli strains used in this study, was used in all experiments ( Fig. 1b and Supplementary Fig. S1 ). At this ampicillin concentration, bacterial cells were non-filamentous (according to microscopy and flow-cytometry analysis), and the population growth was only slightly affected ( Fig. 2a ). We validated the observations made using the reporter fusion by monitoring the cellular amounts of the RpoS and RpoD proteins. Although the amount of RpoD remained stable, the amount of RpoS increased ( Fig. 3 ). Similarly, we also observed an increase in rpoS mRNA levels in ampicillin-treated cells ( Fig. 4 ). In addition to the quantification of the ada mRNA, we also measured the induction of two well-described RpoS-dependent genes, yiaG and fbaB [31] . We found that yiaG and fbaB were 4- and 16-fold induced, respectively, by ampicillin treatment ( Fig. 4 ). Therefore, our data clearly show that the general stress response is induced by subinhibitory concentration of ampicillin in E. coli cells. 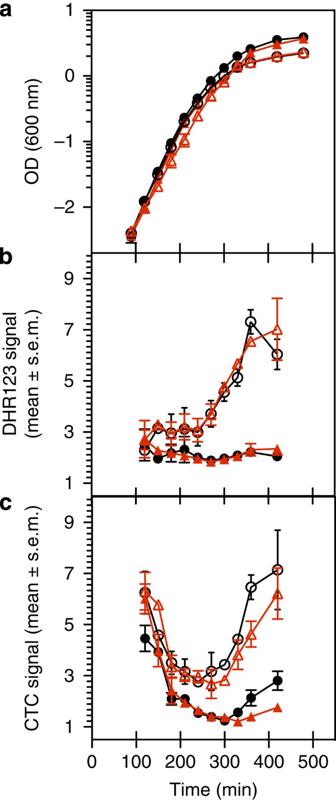Figure 2: Growth and ROS production. Black circles: wild type (wt). Red triangles: ΔrpoS. Filled symbols: untreated controls. Open symbols: treatment with 1 μg ml−1of ampicillin. (a) Growth kinetics were monitored by measuring the optical density at 600 nm. (b) ROS production was measured using fluorescence-activated cell sorting (FACS) and DHR dye. (c) Respiration activity was measured using FACS and CTC dye. For all kinetics, each point represents the mean±s.e.m. of three independent experiments. Figure 2: Growth and ROS production. Black circles: wild type (wt). Red triangles: Δ rpoS . Filled symbols: untreated controls. Open symbols: treatment with 1 μg ml −1 of ampicillin. ( a ) Growth kinetics were monitored by measuring the optical density at 600 nm. ( b ) ROS production was measured using fluorescence-activated cell sorting (FACS) and DHR dye. ( c ) Respiration activity was measured using FACS and CTC dye. For all kinetics, each point represents the mean±s.e.m. of three independent experiments. 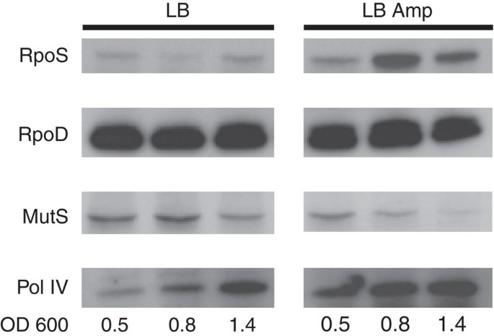Figure 3: Western blot analysis. Western blot analysis of the RpoS, RpoD, MutS and PolIV proteins was performed in cells growing in LB and LB supplemented with 1 μg ml−1of ampicillin (LB Amp). Samples were collected at OD (600 nm) values of 0.5, 08 and 1.4 for both conditions. Total protein loaded was normalized according to nanodrop measurements. Full size image Figure 3: Western blot analysis. Western blot analysis of the RpoS, RpoD, MutS and PolIV proteins was performed in cells growing in LB and LB supplemented with 1 μg ml −1 of ampicillin (LB Amp). Samples were collected at OD (600 nm) values of 0.5, 08 and 1.4 for both conditions. Total protein loaded was normalized according to nanodrop measurements. 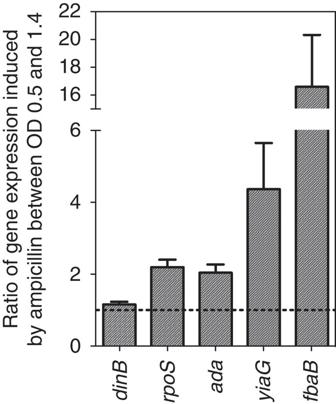Figure 4: mRNA quantification. To quantify levels ofdinB, rpoS, ada, yiaGandfbaBmRNAs, quantitative PCR was performed on cells growing in LB and LB supplemented with 1 μg ml−1of ampicillin. Each point represents the mean±s.e.m. of the ratios of the fold increase relative to the untreated control from three independent experiments. Full size image Figure 4: mRNA quantification. To quantify levels of dinB, rpoS, ada, yiaG and fbaB mRNAs, quantitative PCR was performed on cells growing in LB and LB supplemented with 1 μg ml −1 of ampicillin. Each point represents the mean±s.e.m. of the ratios of the fold increase relative to the untreated control from three independent experiments. Full size image To identify the molecular mechanisms responsible for the induction of the RpoS regulon by a subinhibitory concentration of ampicillin, we used mutants of genes known to be involved in RpoS regulation [18] ( Supplementary Table S2 ). We found that the induction of the RpoS regulon was abolished in a Δ hfq mutant. Hfq is a RNA chaperone that facilitates the post-transcriptional regulation of mRNAs by small RNAs [32] . Several Hfq-dependent small RNAs have been shown to control the rpoS mRNA [18] . We also found that a moderate overexpression of the protease–chaperone complex ClpP–ClpX significantly attenuated this induction ( Fig. 1a ). Because ClpP–ClpX degrades RpoS and is essential for RpoS induction in carbon-starved cells [33] , we speculate that this protease complex is titrated by an increased amount of oxidized and/or denatured proteins in ampicillin-treated cells. Therefore, subinhibitory concentrations of ampicillin increase the cellular amount of the RpoS protein by affecting its induction at the levels of translation and protein stability. Induction of mutagenesis by ampicillin Subinhibitory concentrations of different bactericidal antibiotics, including ampicillin, were previously shown to promote mutagenesis in E. coli [2] , [17] , [24] . Because the RpoS regulon is involved in stress-induced mutagenesis in E. coli [19] , [20] , [34] , we investigated its importance in mutagenesis induced by a subinhibitory concentration of ampicillin using two different mutation assays ( Fig. 5 and Supplementary Fig. S2 ). The first assay scores loss-of-function mutations in the λ cI (Ind − ) repressor gene that represses the tetA gene [35] ( Fig. 5 ). Mutational inactivation of the λ cI (Ind − ) gene confers resistance to tetracycline. The second assay scores gain-of-function mutations in the rpoB gene that confer resistance to rifampicin ( Supplementary Fig. S2 ). The former mutation assay allows the detection of all possible types of mutations, whereas the latter scores mostly base substitutions. For this reason, we used the λ cI (Ind − ) allele to analyse the spectrum of mutations induced by ampicillin treatment ( Supplementary Fig. S3a–c ). We observed an eight-fold higher frequency of tetracycline-resistant mutants (Tet R ) and a three-fold higher frequency of rifampicin-resistant mutants (Rif R ) in populations of the wild-type cells treated with ampicillin compared with an untreated control ( Fig. 5 ; Supplementary Table S2 ). The λ cI (Ind − ) mutation spectrum analysis showed that ampicillin treatment increased the frequency of frameshift mutations and increased the frequency of base substitutions and insertion-sequence mobility to an even greater extent ( Supplementary Fig. S3a–c ). The relative occurrence of different types of mutations induced by ampicillin treatment are as follows: frameshifts represented 52% of the mutations in untreated cells and 20% in treated cells; base substitutions were 35% in untreated cells and 50% in treated cells; and insertion-sequence (IS 1 and IS 5 ) mobility was not detected in untreated cells but represented 17% of the mutations in treated cells. 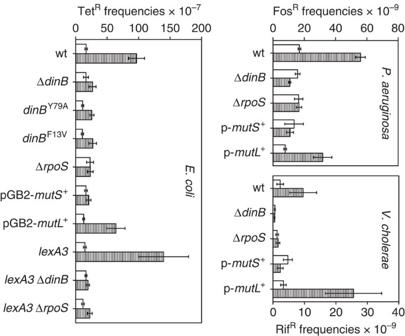Figure 5: β-lactam antibiotic-induced mutagenesis in different bacterial species. Bacteria were grown in LB (open bar) or LB supplemented with the following β-lactam antibiotics (filled bar): 1 μg ml−1of ampicillin, 16 μg ml−1of carbenicillin and 0.5 μg ml−1of ampicillin forE. coli,P. aeruginosaPA14 andV. cholerae, respectively. The frequency of the tetracycline- (TetR), fosfomycin- (FosR) and rifampicin-resistant (RifR) mutants were measured forE. coli,P. aeruginosaPA14 andV. cholerae,respectively. Relevant genotypes are indicated. Each result represents the mean±s.e.m. of at least three independent experiments. wt, wild type. Figure 5: β-lactam antibiotic-induced mutagenesis in different bacterial species. Bacteria were grown in LB (open bar) or LB supplemented with the following β-lactam antibiotics (filled bar): 1 μg ml −1 of ampicillin, 16 μg ml −1 of carbenicillin and 0.5 μg ml −1 of ampicillin for E. coli , P. aeruginosa PA14 and V. cholerae , respectively. The frequency of the tetracycline- (Tet R ), fosfomycin- (Fos R ) and rifampicin-resistant (Rif R ) mutants were measured for E. coli , P. aeruginosa PA14 and V. cholerae, respectively. Relevant genotypes are indicated. Each result represents the mean±s.e.m. of at least three independent experiments. wt, wild type. Full size image ROS production and mutagenesis induced by ampicillin RpoS induction is known to be involved in stress-induced mutagenesis during carbon starvation [19] . Therefore, we measured the involvement of this regulon in ampicillin-induced mutagenesis. We observed no increase in mutagenesis in the Δ rpoS strain using our two mutation assays ( Fig. 5 and Supplementary Fig. S2 ). This result indicates that the induction of the RpoS regulon is essential for ampicillin-induced mutagenesis. It was proposed that the cytotoxic and mutagenic properties of bactericidal antibiotics are direct consequences of the ROS production that results from a perturbation of the TCA cycle [2] , [36] . We evaluated respiratory activity and ROS production in our experimental conditions and determined whether the absence of mutagenesis in the Δ rpoS strain was caused by a decrease in ROS production. We measured the respiratory activity of cells using 5-cyano-2,3-ditolyl tetrazolium chloride (CTC) dye [37] ( Fig. 2c ) and found that it was increased in both the wild-type strain and the Δ rpoS strain. By using dihydrorhodamine 123 (DHR) to detect ROS [38] , we found that the subinhibitory concentration of ampicillin induced the same amount and kinetics of ROS accumulation in the wild-type and Δ rpoS strains ( Fig. 2b ). Therefore, the absence of the ampicillin-induced mutagenesis in the Δ rpoS strain was not due to reduced ROS production. Because RpoS is not involved in the production of ROS in ampicillin-treated cells, we sought to identify RpoS-regulated cellular functions that are required for ampicillin-induced mutagenesis. Involvement of PolIV in ampicillin-induced mutagenesis To investigate in detail how RpoS contributes to ampicillin-induced mutagenesis, we assessed the involvement of the PolIV encoded by the dinB gene. This polymerase is regulated by RpoS and is involved in mutagenesis during prolonged carbon source starvation [20] , [21] . In addition, PolIV is responsible for frameshift mutations in ceftazidime-treated E. coli cells. We used the two previously described assays to measure mutagenesis induced by ampicillin treatment in the Δ dinB strain. Both of the assays indicated that PolIV is required for the mutagenesis induced by subinhibitory concentrations of ampicillin ( Fig. 5 and Supplementary Fig. S2 ). The analysis of cI mutation spectra induced by the subinhibitory concentration of ampicillin showed that PolIV is responsible for the vast majority of ampicillin-induced mutations ( Supplementary Fig. S3a–c ). PolIV can replicate undamaged DNA and is also able to perform translesion synthesis. We tested two dinB alleles, dinB Y79A and dinB F13V , that code for enzymes unable to perform translesion synthesis while retaining the ability to replicate an undamaged template [39] . It was previously shown in vitro that the PolIV F13V protein has a severely reduced ability to incorporate 7,8-dihydro-8-oxoguanine (8-oxo-G) [22] . Because the replacement of the wild-type dinB gene with mutant alleles abolished ampicillin-induced mutagenesis ( Fig. 5 ), it can be concluded that PolIV-generated mutations occur during translesion synthesis and/or by the incorporation of 8-oxo-G. The dinB gene is also regulated by LexA, the repressor of the SOS regulon that is induced by DNA damage and/or replication blockage [40] . SOS induction increases the amount of PolIV from approximately 250–2,500 molecules per cell [41] , and it has also been proposed to be a key factor in the mutagenesis induced by subinhibitory concentrations of antibiotics [2] . Therefore, to test whether the activation of the SOS regulon was required for mutagenesis induced by subinhibitory concentrations of ampicillin, we used a lexA3 (Ind − ) allele that encodes an uncleavable LexA repressor protein [42] . Introduction of the lexA3 (Ind − ) allele in the wild-type strain did not abolish mutagenesis in cells treated with ampicillin ( Fig. 5 ), indicating that the basal expression of LexA-controlled genes was sufficient for ampicillin-induced mutagenesis. Therefore, it is possible that the previously observed involvement of the RecA protein in the mutagenesis of E. coli induced by subinhibitory concentrations of antibiotics [43] was not due to its involvement in the stimulation of the LexA autocleavage but was instead due to some other function of the RecA protein. Inactivation of the dinB or rpoS gene in the lexA3 (Ind − ) background abolished the mutagenesis, as in the lexA wt strain ( Fig. 5 ). Finally, we did not observe induction of the p sulA::gfp reporter gene fusion by subinhibitory concentrations of ampicillin [44] . We also measured the dinB mRNA levels in cells treated with ampicillin, and we found that these levels did not increase compared with those observed in an untreated control ( Fig. 3b ). Hence, the RpoS sigma factor does not induce dinB gene expression in cells treated with a subinhibitory concentration of ampicillin, as has been reported for carbon source-starved stationary-phase cells [20] . It can be concluded that the basal expression of dinB is sufficient for ampicillin-induced mutagenesis. Nonetheless, western blot analysis revealed an increased amount of PolIV protein in treated cells ( Fig. 3 ). It has been shown that the protease–chaperone complex ClpP–ClpX degrades PolIV and thus limits its effect on stress-induced mutagenesis [45] . Consequently, we speculate that the increased amounts of PolIV may result from a titration of ClpP–ClpX, as we have proposed for the RpoS protein above. However, we cannot exclude the participation of an unknown RpoS-regulated molecular intermediate that has an impact on the protein stability of PolIV. Downregulation of the mismatch-repair activity by ampicillin The analysis of the λ cI (Ind − ) spectrum showed large increases in GC→AT and AT→GC transition frequencies: 9.5- and 9-fold, respectively ( Supplementary Fig. S3a ). Because these two transitions are a hallmark of mismatch-repair deficiency [46] , we investigated the involvement of MutL and MutS proteins in the mutagenesis induced by subinhibitory concentrations of ampicillin. MutS is a mismatch-detecting and -binding protein, and MutL acts as a molecular matchmaker between MutS–mismatch complexes and other proteins that help correct replication errors [47] . Importantly, mismatch-repair efficiency is decreased during stationary phase due to the RpoS- and Hfq-dependent depletion of the MutS protein [48] without significant changes in the amount of MutL protein. For this reason, we slightly overproduced the MutS or MutL proteins by introducing low-copy-number plasmids that carry either the mutS or mutL genes. We found that the ampicillin-induced mutagenesis was abolished by MutS protein overproduction but was not significantly affected by the MutL protein overproduction ( Fig. 5 and Supplementary Fig. S2 ). Reciprocally, we confirmed that MutS protein levels decrease in ampicillin-treated cells relative to the levels observed in an untreated control ( Fig. 3 ). Analysis of the cI mutation spectrum showed that the frequency of all ampicillin-induced mutations decreased upon MutS protein overproduction ( Supplementary Fig. S3a–c ). This observation indicated that mismatch-repair overproduction was dominant over the mutagenic potential of the oxidative DNA damage, the PolIV activity level and other error-prone mechanisms. We propose that the fixation of ampicillin-induced mutations is strongly favoured because the mismatch-repair efficiency is reduced by MutS protein depletion. Genetic requirements for the β-lactam-induced mutagenesis in different bacterial species It is difficult to assess the ecological and evolutionary significance of any phenomenon without knowing its distribution in nature. The key factors in the mutagenesis induced by subinhibitory concentration of ampicillin, RpoS, PolIV and mismatch repair are conserved in many bacterial species, but it was unknown whether this phenomenon is unique to E. coli . For this reason, we tested the genetic requirements for mutagenesis induced by subinhibitory concentration of antibiotics in V. cholerae and P. aeruginosa using wild-type dinB and rpoS strains, in addition to strains overproducing the MutS and MutL proteins. The results showed that subinhibitory concentrations of β-lactam antibiotics increased mutagenesis in all tested species and that mutagenesis was abolished, as for E. coli in Δ dinB , Δ rpoS and MutS-overexpressing strains. This demonstrated that the genetic requirement for β-lactam-induced mutagenesis is shared by different bacterial species ( Fig. 5 ). An RpoS-dependent small RNA controls mismatch activity In both exponential and stationary-phase E. coli cells, the expression of the mutS gene is regulated by the Hfq RNA chaperone [48] , indicating the involvement of a small RNA in this regulation. In silico analysis predicted that SdsR small RNA may form a stable RNA duplex with the coding sequence of the mutS mRNA, suggesting that it acts as a post-transcriptional repressor of MutS synthesis. SdsR was recently reported to be under tight positive control of RpoS [49] . The SdsR RNA is conserved in many enterobacterial species and is activated in both stationary-phase cells and growing cells that are subjected to osmotic stress or heat shock [49] . We performed RNA footprinting assays in which 5′-end-labelled SdsR RNA was incubated in the absence or presence of unlabelled mutS m RNA. The incubations were treated with lead(II) acetate ( Fig. 6a ) to induce backbone cleavage of single-stranded RNA. A comparison of the cleavage patterns showed that incubation with target mutS mRNAs resulted in pronounced ‘footprints’ on SdsR RNA ( Fig. 6a , lanes 3 and 4). The protection observed in the presence of mutS mRNA leads us to propose an imperfect >25 bp SdsR– mutS RNA duplex ( Fig. 6c ). To further validate this duplex, we annealed the SdsR and mutS RNA and subjected them to the double-strand-specific RNase III ( Fig. 6b ). Although we observed several weak RNase III cleavages in SdsR RNA alone ( Fig. 6b , lanes 1 and 2), the enzyme strongly and specifically cleaved the SdsR RNA in the mutS complementary region ( Fig. 6 , lanes 3 and 4). Collectively, these results show that the SdsR small RNA can recognize the predicted target region in the mutS mRNA and that the resulting duplex can be cleaved by the house-keeping endonuclease RNase III. 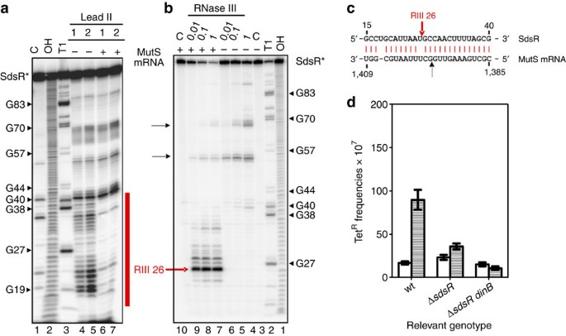Figure 6:In vitroSdsR–mutSmRNA interaction andin vivoeffect ofsdsRinactivation. (a,b) 5′-end-labelled SdsR RNA (~5 nM, SdsR*) treated with lead(II) (a) or RNase III (b) in the absence (lane −) or presence ofmutSmRNA. 5′-end-labelled SdsR RNA was subjected to lead(II) cleavage for 1 or 2 min in the absence (lanes 4 and 5) or presence of coldmutSRNAs (lanes 6 and 7, ~1 μM final). The synthesized target RNA fragment comprises regions +1,222 bases to+1,539 bases downstream of themutSstart codon. Lane C: untreated SdsR RNA. Lane T1: RNase T1 ladder of hydrolysed denatured SdsR RNA. The position of cleaved G residues is given to the left of the gel (a) or to the right of the gel (b). Lane OH: alkaline ladder. Vertical bars indicate the SdsR region protected by mutS RNA. The red arrow denotes specific RNase III cleavage of SdsR in the presence ofmutSmRNA, and the black arrows correspond to RNase III cleavage on SdsR alone. MutS RNA induces strong RNase III cleavage of the SdsR RNA at position U26 (red arrow inb). (c) Proposed RNA duplexes formed by SdsR withmutSmRNAs as derived from the probing results shown ina. Positions in the target sequences are relative to the start of transcription of each RNA. Vertical arrows denote RNase III cleavage of SdsR in complex with target RNAsin vitro. (d) Frequency of ampicillin-induced tetracycline-resistant mutants in the wild-type (wt), ΔsdsRand ΔsdsRΔdinBstrains. Bacteria were grown in LB (open bar) or LB supplemented with 1 μg ml−1of ampicillin (filled bar); each result represents the mean±s.e.m. of at least three independent experiments. Figure 6: In vitro SdsR– mutS mRNA interaction and in vivo effect of sdsR inactivation. ( a , b ) 5′-end-labelled SdsR RNA (~5 nM, SdsR*) treated with lead(II) ( a ) or RNase III ( b ) in the absence (lane −) or presence of mutS mRNA. 5′-end-labelled SdsR RNA was subjected to lead(II) cleavage for 1 or 2 min in the absence (lanes 4 and 5) or presence of cold mutS RNAs (lanes 6 and 7, ~1 μM final). The synthesized target RNA fragment comprises regions +1,222 bases to+1,539 bases downstream of the mutS start codon. Lane C: untreated SdsR RNA. Lane T1: RNase T1 ladder of hydrolysed denatured SdsR RNA. The position of cleaved G residues is given to the left of the gel ( a ) or to the right of the gel ( b ). Lane OH: alkaline ladder. Vertical bars indicate the SdsR region protected by mutS RNA. The red arrow denotes specific RNase III cleavage of SdsR in the presence of mutS mRNA, and the black arrows correspond to RNase III cleavage on SdsR alone. MutS RNA induces strong RNase III cleavage of the SdsR RNA at position U26 (red arrow in b ). ( c ) Proposed RNA duplexes formed by SdsR with mutS mRNAs as derived from the probing results shown in a . Positions in the target sequences are relative to the start of transcription of each RNA. Vertical arrows denote RNase III cleavage of SdsR in complex with target RNAs in vitro . ( d ) Frequency of ampicillin-induced tetracycline-resistant mutants in the wild-type (wt), Δ sdsR and Δ sdsR Δ dinB strains. Bacteria were grown in LB (open bar) or LB supplemented with 1 μg ml −1 of ampicillin (filled bar); each result represents the mean±s.e.m. of at least three independent experiments. Full size image We also tested the genetic requirement of sdsR in the mutagenesis induced by the ampicillin treatment ( Fig. 6d ). We found that the deletion of sdsR did not affect spontaneous mutagenesis but significantly diminished ampicillin-induced mutagenesis. The combination of the sdsR and dinB knockouts completely abolishes ampicillin-induced mutagenesis. These data indicate that the induction of sdsR is an RpoS-dependent function required for ampicillin-induced mutagenesis via its interaction with the mutS mRNA. The capacity of bacteria to resist and adapt to constantly changing environmental conditions depends greatly on a variety of stress responses that enable them to endure negative impacts on fitness and survival [50] . Many bacterial stress responses are regulated by sigma factors that bind to the RNA polymerase core and allow it to initiate transcription at different classes of promoters [50] . The RpoS sigma factor is conserved within gamma-, beta- and delta-proteobacteria [51] and governs the induction of the general stress response that is triggered by many different stresses [18] . In this study, we provide evidence that subinhibitory concentrations of bactericidal antibiotics belonging to different families, such as quinolones, aminoglycosides and β-lactams, induce the RpoS-regulated general stress response in E. coli . We investigated the molecular basis of the RpoS-regulon induction using the β-lactam antibiotic ampicillin as a model drug. We found that ampicillin treatment increases the cellular amount of the RpoS protein by affecting its expression at the levels of translation and protein stability. We also showed that induction of the RpoS regulon is required for the PolIV-dependent mutagenesis induced by subinhibitory concentrations of ampicillin and elucidated the underlying molecular mechanism. It was previously reported that subinhibitory antibiotic treatments increase mutagenesis by perturbing the TCA cycle and, thus, increasing ROS production [2] . We found that the treatment with a subinhibitory concentration of ampicillin increases the intracellular amount of ROS to the same level observed in the wild-type and Δ rpoS strains. Therefore, the ampicillin-induced mutagenesis cannot simply be due to more mutagenic oxidative damage in the wild-type relative to the rpoS strain. This finding indicates that some of the RpoS-regulated cellular functions are required for the ampicillin-induced mutagenesis. RpoS was reported to be involved in the control of dinB gene expression and PolIV-mediated mutagenesis [20] , [21] . However, we found that dinB gene expression was not increased by the ampicillin treatment. This result corroborates the previously published observation that RpoS does not regulate dinB gene induction in ampicillin-treated cells [24] . The comparison of the λ cI (Ind − ) mutation spectra of wild-type and dinB strains showed that PolIV is responsible for the generation of the vast majority of ampicillin-induced mutations. This DNA polymerase generates mostly frameshifts in vitro and in vivo in strains that overexpress the dinB gene [52] , [53] . However, we found that PolIV generates more base substitutions than frameshifts in ampicillin-treated cells. A similar predominance of base-substitution mutations was also observed in a study in which PolIV was under control of its native promoter and the mutational target was a chromosomal locus, as in our study [54] . Because base substitutions are more likely to result in new gene function and frameshifts generally inactivate genes, the spectrum of PolIV-generated mutations in ampicillin-treated cells could be relevant to the evolution of antibiotic resistance. The largest increases in the PolIV-dependent ampicillin-induced base substitutions were GC→AT and AT→GC transitions and AT→CG transversions. AT→CG transversions usually result from the incorporation of 8-oxo-G during DNA replication [55] . The increase in these transversions is in full agreement with data from other laboratories showing that the lethality of β-lactam and other bactericidal antibiotics requires PolIV that is able to incorporate oxidized nucleotides into newly synthesized DNA [22] . Large increases in GC→AT and AT→GC transitions are usually a hallmark of a mismatch-repair deficiency [46] . We showed that although these mutations are generated by PolIV, they are fixed because mismatch-repair activity diminishes in ampicillin-treated cells. Mismatch-repair efficiency in ampicillin-treated cells is reduced as a consequence of MutS protein depletion. It was previously observed that the intracellular amount of the MutS protein decreases in stationary-phase E. coli cells by an Hfq- and RpoS-dependent mechanism [48] . Although mismatch-repair deficiency may not affect cells that are not actively growing, it causes increased mutagenesis in growing cells, as we have shown in our study. We also present data to suggest that the RpoS- and Hfq-controlled small RNA SdsR [49] may directly repress the mutS mRNA by forming a >25 nucleotide RNA duplex with this messenger. Based on our observation that inactivation of the sdsR gene abolishes ampicillin-induced mutagenesis, we propose that the RpoS-dependent SdsR induction is responsible for the reduction in MutS levels in ampicillin-treated cells. This MutS depletion leads to diminished control over DNA-replication fidelity and, ultimately, leads to increased mutagenesis. It is important to note that mismatch repair corrects errors of the replicative DNA polymerase and also of PolIV [52] , which can explain why MutS overproduction abolished the ampicillin-induced mutagenesis in the rpoS + dinB + background. It is also important to note that β-lactam-induced mutagenesis is controlled by the RpoS, PolIV and MutS-limitation-dependent pathway in the two other bacterial species examined in this study, V. cholerae and P. aeruginosa. Whether these bacteria possess SdsR-like small RNAs remains to be determined. Mutator phenotypes have been associated with the generation of antibiotic resistance in many bacterial species [56] , [57] , [58] . In this study, we provide evidence that bacteria possess molecular mechanisms allowing them to adapt mutation rates to environmental conditions. The RpoS-dependant downregulation of the mismatch-repair efficiency does not improve resistance to stressors, but by increasing the mutation frequency, it increases the probability of generating adaptive mutations. Given that this cellular response is induced in many different bacteria and by many different stresses, including antibiotics, this mechanism may have a major role in bacterial adaptive evolution in general and in the generation of resistance to antibiotics in particular. Bacterial strains and growth conditions Bacterial strains used in this study are described in Supplementary Table S3 . All E. coli strains were derived from the MG1655 strain. The PadaZ and MGCI strains were used as reference strains to measure RpoS-regulon induction and mutant frequencies, respectively. Allelic transductions from the Keio or INSERM laboratory collections to reference strains were performed using classical P1 vir transduction. Other E. coli mutant constructions are described in the Supplementary Methods . All V. cholerae strains were derived from the V. cholerae N16961 hapR + El tor strain, which is considered to be a V. cholerae reference strain. The methods used to generate the V. cholerae mutants are described in the Supplementary Methods . All P. aeruginosa strains are derived from the PA14 strain, which is considered to be a P. aeruginosa reference strain. Liquid cultures were grown in large Erlenmeyer flasks with a ratio of 90% air to 10% liquid LB medium (Difco) at 37 °C with shaking at 200 r.p.m. LB agar (Difco) plates were also incubated at 37 °C. When needed, media was supplemented with the appropriate antibiotic concentrations. Determination of the minimal inhibitory concentration For E. coli, the MIC was defined as the antibiotic concentration that inhibited growth after 24 h of incubation in LB liquid medium at 37 °C. Cells from fresh overnight cultures were diluted 1/100,000 v/v and inoculated into 96-well microtiter plates containing LB and antibiotics. Microtiter plates were incubated for 24 h at 37 °C in a microplate reader and incubator (IEMS reader system from Labsystems). The optical density at 600 nm was measured every 5 min. The MIC was determined to be 2 μg ml −1 . For V. cholerae , the MIC was determined using E-tests and was determined to be 1 μg ml −1 . The P. aeruginosa carbenicillin MIC was determined by the microdilution method, as recommended by the Clinical and Laboratory Standards Institute, but LB medium was used instead of Müller–Hinton. Screening for the induction of p ada :: lacZ by antibiotics Screening was performed using a standard disc diffusion assay. Stationary-phase cultures were diluted 1/100 in TA medium (Difco) containing X-Gal. A 5 ml aliquot of the inoculated TA medium was spread onto an LB agar plate containing X-Gal. A single disc of Whatman paper was placed on each plate, and antibiotics or chemicals were added to the disc. The plates were incubated overnight at 37 °C in the dark. β-galactosidase activity assay β-galactosidase activity was determined as described by Miller. A pellet of cells from 1 ml of culture was resuspended in Z-buffer (NA 2 HPO 4 16.1 g l −1 , NaH 2 PO 4 5.5 g l −1 , KCl 0.75 g l −1 , MgSO 4 0.246 g l −1 and β-mercaptoethanol 0.3% v/v ). Cells were lysed with 20 μl of chloroform and 10 μl of 0.1% SDS. The reaction was started at 30 °C by adding 200 μl of ONPG (4 g ml −1 ), and it was stopped by the addition of 500 μl of NaCO 3 solution (pH 9). β-galactosidase activity was expressed as Miller units. Mutation assays For E. coli and V . cholerae , cells from fresh overnight cultures were inoculated (1/100,000) into plain LB medium or LB medium containing 1 μg ml −1 of ampicillin for E. coli , and 0.5 μg ml −1 for V. cholerae , which corresponds to 50% of the MIC of ampicillin, and incubated for 10 h at 37 °C at 200 r.p.m. in the dark. Appropriate dilutions of cells were spread on the LB plate containing 100 μg ml −1 of rifampicin or 12.5 μg ml −1 of tetracycline. The total number of CFUs was determined on LB agar plates. Colonies were scored after 2 days of incubation at 37 °C. For P. aeruginosa , 10 5 cells from an overnight culture were inoculated in 3 ml of plain LB or LB containing 16 μg ml −1 of carbenicillin, which corresponds to 50% of the MIC of carbenicillin, and allowed to grow for 6 h. The cells were then washed with LB and allowed to recover for 14 h. The total CFUs were determined on LB agar plates, and fosfomycin-resistant mutants were determined by plating the appropriate dilution on LB plates containing fosfomycin (128 μg ml −1 ). Spectrum of mutations that inactivate the cI gene The mutation spectrum induced by the treatment with a subinhibitory concentration of ampicillin was determined by sequencing the 1122 nucleotide-long PCR product of the cis (promoter region) and the trans -regulatory ( cI gene) region that controls the expression of the tetA gene. Cells were treated as for the mutagenesis measurements described above. A total of 100 randomly chosen Tet R mutants per genotype and per condition were isolated and used for the PCR amplification using the following primers: P1: 5′-TCAGCCAAACGTCTCTTCAG-3′ and P2: 5′-GCCAATCCCCATGGCATCGAGTAAC-3′. Fluorescence-activated cell sorting E. coli cells were treated as for the mutagenesis measurements described above. Cells were collected every 30 min. After measuring the optical density at 600 nm, cells were incubated for 30 min in the dark at 4 °C in PBS (pH 7.4) containing 1 mM DHR (Sigma) or 5 mM CTC [37] . Fluorescent profiles were measured for DHR at 488 nm excitation and 530 nm emission and for CTC at 488 nm excitation and 670 nm emission. A minimum of 50,000 cells was analysed for each time point with a maximum of 2,000 events counted per second. Western blot analysis E. coli cells were treated as for the mutagenesis measurement described above. Cells were collected at the indicated optical densities. Proteins were extracted using Novagen BugBuster lysis buffer and the addition of 5 U ml −1 of Benzonase. Approximately 50–200 μg of protein was resolved on a 4–20% polyacrylamide gradient gel (Bio-Rad). Proteins were then transferred to a polyvinylidene difluoride membrane. Antibodies used for this study include anti-RpoS (rabbit [59] ) 1/150,000 em , rabbit anti-MutS (Genecheck) 0.2 μg ml −1 , anti-DinB (rabbit) 1/500 em , anti-RpoD (mouse; Abcam) 1/10,000, anti-IgG-mouse (goat; Neoclone) 1/10,000 and anti-IgG-rabbit (mouse; Invitrogen) 1/50,000. Quantitative RT–PCR E. coli cells were treated as for the mutagenesis measurement described above. Cells were collected at the indicated optical densities. RNA was extracted using the RNA prep kit (Macherey Nalgene) and a Turbo DNase (Ambion) treatment. A minimum of 2 μg of RNA was used for the synthesis of cDNA using Superscript III (Invitrogen). Quantitative PCR was performed using the SYBRgreen method [60] . Primers used in this study are listed in Supplementary Table S4 . In vitro transcription and 5′-end labelling Chemicals and reagents were purchased from Sigma-Aldrich or GE Healthcare unless otherwise specified. Oligodeoxyribonucleotides were obtained from Sigma-Genosys ( Supplementary Table S5 ). DNA templates carrying a T7 promoter sequence for in vitro transcription were generated by PCR using genomic DNA (E. coli K12 strain). The primers used to generate templates for the transcription of mutS mRNA and SdsR are listed in Supplementary Table S1 . RNA was transcribed in vitro using the MEGAscript High Yield Transcription Kit (Ambion, no. 1333) followed by DNase I digestion (1 U, 15 min, 37 °C). Following phenol extraction, the RNA was purified on a G25 column to remove unincorporated ribonucleoside triphosphates and was then precipitated with ethanol. The RNA integrity was checked on a denaturing polyacrylamide gel. For 5′-end labelling, 20 pmol of in vitro synthesized RNA was dephosphorylated with 10 U of calf intestinal alkaline phosphatase (New England Biolabs) for 1 h at 37 °C. Following organic extraction and precipitation, the RNA was 5'-end labelled with 32 P-γATP (20 μCi) with 1 U of polynucleotide kinase (New England Biolabs) for 30 min at 37 °C. Unincorporated nucleotides were removed as described above, and the RNA was purified on a denaturing PAA gel. Upon visualization on a phosphorimager, the RNA was excised from the gel and eluted overnight in elution buffer (0.1 M sodium acetate, 0.1% SDS and 10 mM EDTA) at 4 °C followed by organic extraction and precipitation RNA secondary structure probing Secondary structure probing and mapping of RNA complexes was conducted on 5′-end-labelled RNA (~0.1 pmol) in a total volume of 10 μl. The RNA was denatured for 1 min at 95 °C and chilled on ice for 5 min before the addition of 1 μg yeast RNA (Ambion) and 10 × structure buffer (0.1 M Tris pH 7, 1 M KCl and 0.1 M MgCl 2 ; Ambion). Denatured, unlabelled sRNA/mRNA fragment was added in excess amounts, as indicated in the figure legends. After incubation for 10 min at 37 °C, 2 μl of a fresh solution of lead(II) acetate (25 mM; Fluka no. 15319) was added, and the reaction was incubated for 1 or 2 min at 37 °C, respectively. To map the RNase III (Ambion) cleavage sites, RNA complexes were formed as above, except for the addition of 1 mM DTT to the reactions. Incubations were conducted at 37 °C for 5 min after the addition of RNase III (1, 0.1 or 0.01 U) before stopping the reactions. The reactions were stopped by adding 5 μl of 0.1 M EDTA, precipitating and dissolving in loading buffer II (95% formamide, 18 mM EDTA, 0.025% SDS, xylene cyanol and bromophenol blue; Ambion) or by the direct addition of 12 μl loading buffer on ice. RNase T1 ladders were obtained by incubating labelled RNA (~0.2 pmol) in 1 × sequencing buffer (Ambion) for 1 min at 95 °C. Subsequently, 1 μl of RNase T1 (0.1 U μl −1 ) was added and the incubation continued at 37 °C for 5 min. OH ladders were generated by incubating 0.2 pmol of labelled RNA in alkaline hydrolysis buffer (Ambion) at 95 °C for 5 min. Reactions were stopped with 12 μl loading buffer. Samples were denatured for 3 min at 95 °C before separation on 6% polyacrylamide/7 M urea sequencing gels in 1 × TBE. The gels were dried and analysed using a PhosphorImager (Molecular Dynamics). How to cite this article: Gutierrez, A. et al . β-lactam antibiotics promote bacterial mutagenesis via an RpoS-mediated reduction in replication fidelity. Nat. Commun. 4:1610 doi: 10.1038/ncomms2607 (2013).